A TAL effector repeat architecture for frameshift binding Transcription activator-like effectors (TALEs) are important Xanthomonas virulence factors that bind DNA via a unique tandem 34-amino-acid repeat domain to induce expression of plant genes. So far, TALE repeats are described to bind as a consecutive array to a consecutive DNA sequence, in which each repeat independently recognizes a single DNA base. This modular protein architecture enables the design of any desired DNA-binding specificity for biotechnology applications. Here we report that natural TALE repeats of unusual amino-acid sequence length break the strict one repeat-to-one base pair binding mode and introduce a local flexibility to TALE–DNA binding. This flexibility allows TALEs and TALE nucleases to recognize target sequence variants with single nucleotide deletions. The flexibility also allows TALEs to activate transcription at allelic promoters that otherwise confer resistance to the host plant. Transcription activator-like effectors (TALEs) employ a programmable DNA-binding domain and have revolutionized biotechnology approaches that use sequence-specific DNA-binding proteins [1] , [2] , [3] . Natural TALEs are injected by plant pathogenic Xanthomonas spp. bacteria via a type-III secretion system into plant cells [4] . Inside the plant cell they function as transcription factors that activate target gene expression and support bacterial colonization [2] , [5] . TALEs contain a unique DNA-binding domain of tandem near-identical 34-amino-acid repeats. The repeats are highly conserved and mainly differ in two adjacent amino acids (positions 12 and 13) termed repeat-variable diresidue (RVD) [5] , [6] . In the array each repeat recognizes one nucleotide in the target DNA sequence, and the RVD specifies which base is bound [6] , [7] . In addition to the repeat region, the N-terminal part of TALEs contains four degenerated repeats (termed repeat 0, −1, −2 and −3) that contribute to DNA-binding [8] . Repeat −1 specifies thymine that typically precedes TALE target sequences [7] , [9] , [10] . The C-terminal part of TALEs contains two functional nuclear localization signals as well as an acidic activation domain that is important for gene activation [4] , [11] . Xanthomonas oryzae pv. oryzae ( Xoo ) and Xanthomonas oryzae pv. oryzicola ( Xoc ) cause bacterial leaf blight and bacterial leaf streak, respectively, which are two of the most devastating diseases of the staple crop rice [12] , [13] . Both pathogens contain a particularly large number (7–28) of TALE genes per strain [14] and the TALE-dependent modulation of host gene expression profiles is an important feature of Xoo and Xoc diseases. In some cases, loss of a single TALE gene severely compromised bacterial virulence [5] . The best-studied group of TALE virulence targets is the SWEET gene family in rice. Three members of this gene family are targets of several TALEs from different Xoo strains. OsSWEET11 and OsSWEET13 are targeted by PthXo1 and probably PthXo2, respectively, whereas OsSWEET14 is targeted by four different TALEs, TalC, AvrXa7, PthXo3 and TAL5, originating from different Xoo strains [15] , [16] , [17] , [18] , [19] , [20] , [21] . Furthermore, it was shown that OsSWEET12 , OsSWEET13 and OsSWEET15 support bacterial colonization if induced by designer TALEs [16] , [19] . Considering that >100 Xanthomonas TALEs are known the overall number of identified plant target genes is low. One approach to overcome this is by using computational algorithms to predict possible TALE targets [22] , [23] , [24] . Using the TALE RVD–DNA code the promoter sequences of host plants are scanned for potential TALE target sites. Promising target candidates contain a TALE target site and are TALE-dependently activated [23] , [24] . Plants have evolved resistances that are based on TALE-dependent activation of genes that trigger a resistance response towards Xanthomonas strains delivering the matching TALE [25] , [26] , [27] . A different resistance mechanism is based on mutation of potential TALE target DNA sequences [17] , [20] , [28] , [29] . These mutations can render virulence targets non-responsive to TALEs, thereby efficiently preventing the contribution of a given TALE to bacterial virulence. If target gene upregulation is important for virulence of the pathogen, the plants become resistant. Accordingly, rice varieties carrying insertions, deletions or substitutions in the promoter sequences of OsSWEET11 and OsSWEET12 are not susceptible to Xoo strains carrying the TALEs PthXo1 and PthXo2, respectively [15] , [17] , [28] , [29] , [30] . The modular TALE architecture allows a free combination of repeats to generate any desired DNA-binding specificity [7] , [31] , [32] . This flexibility resulted in adoption of the TALE repeats as specific DNA-binding domain that can be fused to executor domains to generate different biotechnological tools [2] . The most widespread use is based on fusions of TALEs with a nuclease domain (termed TALEN) to edit eukaryotic genomes at specific sites [3] , [31] , [33] , [34] . Other executor domains were applied for gene activation, gene repression, chromatin modification, fluorescent tagging of chromosomal loci and chromatin affinity purification [35] , [36] , [37] , [38] , [39] , [40] . The three-dimensional (3D) structures of TALE–DNA complexes have been solved [8] , [9] , [10] , [41] . TALE repeats form a right-handed superhelix that wraps around the DNA double strand. The helix–loop–helix structure of a single repeat exposes the RVD amino acid at position 13 to interact with a leading strand base from the DNA major groove. In contrast, the RVD amino acid at position 12 stabilizes the RVD loop by interaction with the carbonyl of position 8 of the same repeat [9] , [10] , [41] . This highly regular repeat architecture is likely necessary to position consecutive repeats correctly to a continuous string of DNA bases. The 3D structures show that in a TALE repeat non-RVD amino acids mediate inter- and intra-repeat interactions as well as connections to the DNA phosphate backbone. This probably supports the correct positioning of the repeat array to the DNA [9] , [10] , [41] . The TALE 3D structures also suggest that significant changes in the repeat length may have a profound impact on DNA binding. Two fairly common exceptions to the typical 34-amino-acid length of TALE repeats exist. These are either 33-amino-acid repeats that have a deletion of the RVD amino acid 13 or 35-amino-acid repeats containing a proline following amino acid 32. In both cases the DNA-binding specificity of TALEs is not altered [7] , [36] , [42] . Thirty-five-amino-acid repeats are also typical in TALE homologues from Ralstonia solanacearum for which a RVD-guided DNA-binding activity analogous to Xanthomonas TALEs was shown [43] , [44] . Interestingly, some naturally occurring Xanthomonas TALEs possess a single repeat of aberrant length besides the canonical 33–35-amino-acid repeats [5] , [45] . These aberrant repeats consist of 30 amino acids (with a 4-amino-acid deletion in the second helix of the repeat), 39 or 40 amino acids (duplication in the second helix of the repeat), or 42 amino acids (duplication in the first helix of the repeat) [5] . It is not known how repeats that differ in length from the normal 33–35 amino acids influence the DNA-binding behaviour of TALEs. Here we analyse how the insertion of a repeat of aberrant length in the canonical repeat array influences TALE function. We find that such TALEs exhibit two possible binding conformations, the normal one and a novel one that tolerates single nucleotide deletions in the target sequence. We show that this binding behaviour expands the recognition specificity of TALEs and TALENs, respectively. Furthermore, we find that the flexible TALE-binding behaviour provides a potential evolutionary solution for Xanthomonas to overcome plant resistance. Natural TALEs with aberrant repeats AvrXa7 and PthXo3 are natural TALEs from Xoo with 25.5 and 28.5 repeats, respectively, that both contain one aberrant repeat of 39 amino acids approximately in the middle of the repeat array ( Fig. 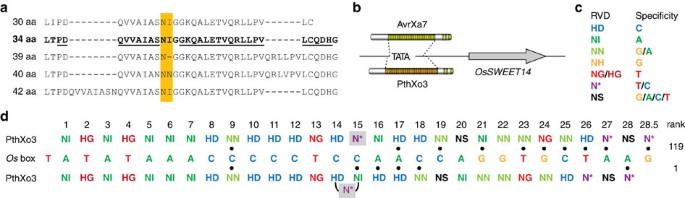Figure 1:Aberrant repeat length variants fromXanthomonasspp. TALEs. (a) Alignment of amino acid (aa) sequences of natural TALE repeats with different length. The repeat-variable diresidues (RVDs) are boxed in yellow. A typical 34-aa repeat is in bold face and the residues forming the two α-helices are underlined. (b) Cartoon of AvrXa7 and PthXo3 binding to their overlapping target sequences at the TATA-box in theOsSWEET14(Os11g31190) promoter. (c) TALE RVDs and their DNA base specificities. (d) PthXo3 RVDs with the aberrant repeat in normal or looped-out conformation aligned to theOsSWEET14promoter target sequence (Osbox). A dot indicates a non-matching RVD–base combination. The rank of both alignments in a target site prediction is indicated. 1 ; Supplementary Figs 1 and 2 and Supplementary Table 1 ). Both TALEs are important virulence factors that support growth of Xoo strains on rice [15] , which demonstrates that they are functional. Indeed, both TALEs induce expression of the rice sugar exporter OsSWEET14 by binding to overlapping target boxes ( Fig. 1b and Supplementary Figs 1 and 2 ) [15] , [18] , [19] . In contrast, computational predictions of AvrXa7 and PthXo3 target sequences rank the PthXo3 site in the OsSWEET14 promoter at position 119 (ref. 23 ). We noticed a high number of non-matching RVD base combinations in the 3′ part of the PthXo3 target box following the aberrant repeat ( Fig. 1c,d and Supplementary Fig. 2 ). If the C-terminal half of the repeat array is shifted one nucleotide upstream by looping out the long repeat, the PthXo3 target box in OsSWEET14 will rank at position 1 in target predictions ( Fig. 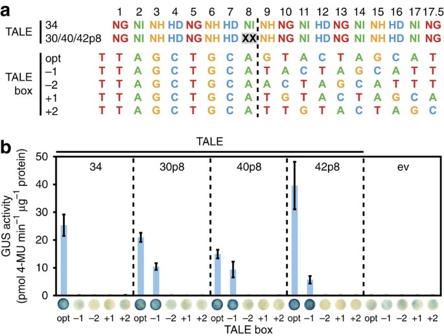Figure 2: Aberrant repeats allow a flexible recognition of target DNA sequences with a −1 nucleotide frameshift. (a) RVDs of artificial TALEs and target boxes. A TALE with all 34-aa repeats or TALEs with an aberrant 30-aa NI-repeat, 40-aa NN-repeat and 42-aa NI-repeat, respectively, at position 8 are constructed. An optimal target box (opt) and derivatives with deletions or insertions of one or two nucleotides (− or +1 or 2) after position 8 (dashed line) are fused to a minimal promoter and a promoter-less GUS reporter gene. (b) GUS assays of TALEs and reporter constructs (n=3). 35S-driven GFP expression serves as empty vector (ev) control in quantitative and qualitative assays. Error bars indicate the s.d. in the quantitative assay. One representative leaf disk of the qualitative assay is shown. 1c and Supplementary Table 2 ; ref. 23 ). Figure 1: Aberrant repeat length variants from Xanthomonas spp. TALEs. ( a ) Alignment of amino acid (aa) sequences of natural TALE repeats with different length. The repeat-variable diresidues (RVDs) are boxed in yellow. A typical 34-aa repeat is in bold face and the residues forming the two α-helices are underlined. ( b ) Cartoon of AvrXa7 and PthXo3 binding to their overlapping target sequences at the TATA-box in the OsSWEET14 ( Os11g31190 ) promoter. ( c ) TALE RVDs and their DNA base specificities. ( d ) PthXo3 RVDs with the aberrant repeat in normal or looped-out conformation aligned to the OsSWEET14 promoter target sequence ( Os box). A dot indicates a non-matching RVD–base combination. The rank of both alignments in a target site prediction is indicated. Full size image To test the recognition specificities of AvrXa7 and PthXo3, we build reporter constructs with an optimal target box according to the TALE specificity code, and derivatives with nucleotide deletions (−1, −2) or insertions (+1, +2) at the nucleotide position behind the one corresponding to the aberrant repeat, respectively ( Supplementary Figs 1a and 2a ). The boxes are inserted upstream of a minimal promoter that has no basal activity [7] . In addition, reporter constructs with either the natural box of AvrXa7 in front of the minimal promoter or the OsSWEET14 promoter fragment containing the natural AvrXa7/PthXo3 box are used ( Supplementary Figs 1a and 2a , ref. 21 ). The reporter constructs are then co-transformed with expression constructs of AvrXa7 or PthXo3 using Agrobacterium into leaves of Nicotiana benthamiana plants. β-glucuronidase (GUS) assays reveal that both TALEs induce expression of the reporter containing either one of the target boxes although they exhibit several non-matching RVD–base combinations ( Supplementary Figs 1b–g and 2b–h ). Possible explanations for this surprising result are that AvrXa7 and PthXo3 contain a large number of repeats, several RVDs with broad specificity like NS, NN and N*, and one repeat of aberrant length. We aim to test the role of the aberrant repeat in a more controlled TALE design. Aberrant repeats permit a novel TALE–DNA-recognition mode We construct artificial TALEs [46] with a 17.5-repeat array that is designed to result in a maximum of non-matching RVD–base combinations upon a possible frameshift in the target sequence. TALEs are assembled with and without single aberrant repeats of 30-, 40- and 42-amino-acid length at position 8 ( Figs 1a and 2a and Supplementary Table 1 ), and analysed in planta for the activation of GUS reporters with optimal and frameshift (−1, −2, +1 and +2) target boxes ( Fig. 2a,b ). The aberrant repeat sequences including their RVDs correspond to the natural X. oryzae TALE sequences ( Supplementary Table 1 ). Figure 2: Aberrant repeats allow a flexible recognition of target DNA sequences with a −1 nucleotide frameshift. ( a ) RVDs of artificial TALEs and target boxes. A TALE with all 34-aa repeats or TALEs with an aberrant 30-aa NI-repeat, 40-aa NN-repeat and 42-aa NI-repeat, respectively, at position 8 are constructed. An optimal target box (opt) and derivatives with deletions or insertions of one or two nucleotides (− or +1 or 2) after position 8 (dashed line) are fused to a minimal promoter and a promoter-less GUS reporter gene. ( b ) GUS assays of TALEs and reporter constructs ( n =3). 35S-driven GFP expression serves as empty vector (ev) control in quantitative and qualitative assays. Error bars indicate the s.d. in the quantitative assay. One representative leaf disk of the qualitative assay is shown. Full size image TALEs with or without an aberrant repeat trigger GUS activity with the reporter construct containing the optimal box. This indicates that all TALEs tested recognize the optimal box and that aberrant repeats function similarly to normal ones in a repeat array. Significantly, only TALEs with an aberrant repeat result also in strong GUS activity with reporter constructs containing the −1 box ( Fig. 2b ). The same effect is apparent in artificial TALEs with a different repeat composition ( Supplementary Fig. 3 ). Thus, a TALE containing exclusively canonical 34-amino-acid repeats is not able to recognize a −1 box, because of many (in this case nine) non-matching RVD–base combinations in either the front or rear part of the box, depending on how the TALE RVDs are aligned to the box. In contrast, a TALE with an aberrant repeat efficiently activates the reporter. These data suggest that an aberrant repeat confers a flexible binding to TALEs. Interestingly, this flexible binding mode is possible with different aberrant repeats that are shorter (30 amino acids) or longer (39, 42 amino acids). The −2, +1 and +2 boxes are not recognized by any of the TALEs, indicating that other binding modes are not supported. Aberrant repeats function at different repeat array positions As in nature single aberrant repeats are positioned more or less in the central region of the repeat array ( Supplementary Table 1 ), we investigate whether TALEs tolerate only this arrangement. We insert the aberrant 40-amino-acid repeat at different positions (positions 3, 8 or 14) in the previously used 17.5 TALE repeat array that is highly susceptible to frameshift in its target sequence ( Fig. 3a ). As target boxes we use either the optimal one or sequences with frameshift at positions 4, 9 and 15, respectively ( Fig. 3a ). GUS reporter assays reveal that TALEs that carry the aberrant repeat at any of the three positions are functional. All TALEs with aberrant repeats recognize the optimal box and the one with a frameshift following the position corresponding to the aberrant repeat in the TALE ( Fig. 3b ). However, the TALE with an aberrant repeat at position 14 displays only weak activity on both the optimal and the corresponding −1 frameshift box ( Fig. 3b ). This suggests that it is not favourable for the overall activity of TALEs if only a small number of repeats (in this case four) follow an aberrant repeat in the array. 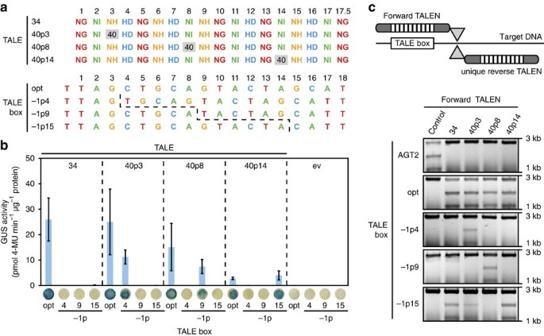Figure 3: Aberrant repeats function at different positions in the repeat array of TALEs and TALENs. (a) TALE RVDs and target boxes. Artificial TALEs or TALENs are constructed with all 34-aa repeats or an aberrant 40-aa NN-repeat inserted at position 3 (40p3), position 8 (40p8) or position 14 (40p14). The NN-repeat recognizes both G and A DNA bases. The boxes are either perfectly matching the specificity of normal repeats (opt) or have one base pair deleted to the right of the dashed line at position 4 (−1p4), position 9 (−1p9) or position 15 (−1p15). (b) GUS assays of TALEs and reporter constructs (n=3). 35S-driven GFP expression serves as empty vector (ev) control in quantitative and qualitative assays. Error bars indicate the s.d. in the quantitative assay. One representative leaf disk of the qualitative assay is shown. (c) Cartoon of TALENs bound to DNA andin vitroTALEN restriction assay. The TALEN pairs are placed such that the FokI domain (grey triangle) can dimerize and cut the DNA. The unique reverse TALEN is constant in all assays. The control TALEN recognizes a different target box (AGT2). Target DNA is incubated within vitro-transcribed and translated TALEN pairs. Restriction fragments are documented on agarose gels. Figure 3: Aberrant repeats function at different positions in the repeat array of TALEs and TALENs. ( a ) TALE RVDs and target boxes. Artificial TALEs or TALENs are constructed with all 34-aa repeats or an aberrant 40-aa NN-repeat inserted at position 3 (40p3), position 8 (40p8) or position 14 (40p14). The NN-repeat recognizes both G and A DNA bases. The boxes are either perfectly matching the specificity of normal repeats (opt) or have one base pair deleted to the right of the dashed line at position 4 (−1p4), position 9 (−1p9) or position 15 (−1p15). ( b ) GUS assays of TALEs and reporter constructs ( n =3). 35S-driven GFP expression serves as empty vector (ev) control in quantitative and qualitative assays. Error bars indicate the s.d. in the quantitative assay. One representative leaf disk of the qualitative assay is shown. ( c ) Cartoon of TALENs bound to DNA and in vitro TALEN restriction assay. The TALEN pairs are placed such that the FokI domain (grey triangle) can dimerize and cut the DNA. The unique reverse TALEN is constant in all assays. The control TALEN recognizes a different target box (AGT2). Target DNA is incubated with in vitro -transcribed and translated TALEN pairs. Restriction fragments are documented on agarose gels. Full size image Flexible TALENs with aberrant repeats TALENs have become state-of-the-art tools for genome editing [3] . TALENs are TALE–DNA-binding domain fusions to the Fok I endonucleolytic domain, which act in pairs to enable Fok I dimerization and DNA cleavage [3] . We test whether aberrant repeats can change the DNA recognition behaviour of TALENs. TALENs with and without an aberrant repeat are assembled. The aberrant 40-amino acid repeat is placed at positions 3, 8 and 14, respectively, in a TALEN of 17.5 repeats ( Fig. 3a ). These ‘forward’ placed TALENs are combined with a common ‘reverse’ placed TALEN with 34-amino-acid repeats ( Fig. 3c and Supplementary Fig. 4b ) and linear DNA fragments containing the target boxes in in vitro restriction assays. The optimal box is cleaved using TALENs with or without an aberrant repeat emphasizing that the normal binding mode is also supported in TALEN assays. In contrast, the boxes with −1 frameshift at position 4 and 9 are only cleaved in the presence of the TALENs with an aberrant repeat at position 3 and 8, respectively ( Fig. 3c and Supplementary Fig. 5 ). This is in accordance with our observation for TALEs before ( Fig. 3b ) that aberrant repeats infer a local flexibility to the repeat array. In contrast, the box with the −1 frameshift at position 15 is recognized not only by the TALEN with an aberrant repeat at position 14 but also by the normal all 34-amino-acid repeat TALEN, and to a lesser degree by the TALEN with an aberrant repeat at position 3. Apparently, these TALENs tolerate three non-matching RVD–base combinations at the end of the repeat array ( Fig. 3c ). This mismatch tolerance of rear repeats in TALENs was not observed in the previous experiments using TALEs in reporter gene activation assays ( Fig. 3b ). It suggests that binding of the rear TALE repeats to DNA is less important for dimerization of the nuclease domains than for function of the natural activation domain. Furthermore, we test whether the TALEN with the aberrant 40-amino-acid repeat at position 8 can perform cleavage of −2, +1 or +2 frameshift boxes ( Supplementary Fig. 4 ). We observe that the TALENs with or without the long repeat do not exhibit activity on these boxes ( Supplementary Fig. 4c ), suggesting that other binding modes are not supported by TALENs similarly to our observation for TALEs ( Fig. 2 ). In summary, our experiments demonstrate that aberrant repeats initiate a flexible DNA-binding behaviour in vivo and in vitro , and that they can be used to expand the recognition specificities of artificial TALEs as well as TALENs. The aberrant repeat is excluded from the interaction So far, it is not clear which repeat of the repeat array is excluded from the interaction, for example by looping out. Our results allow several possible explanations: either the aberrant repeat itself is excluded or the repeat up- or downstream of the aberrant repeat. Therefore, we test TALEs with aberrant repeats at position 8 combined with target boxes (−1) deleted in either the nucleotide at position 7, 8 or 9 in GUS reporter assays ( Fig. 4a ). We expect that the TALE will yield the highest reporter activity in combination with the −1 box that has the deletion exactly in opposite to the repeat that is excluded, because the other boxes will produce at least one non-matching RVD–base combination. Indeed, the target sequence with the nucleotide deleted at position 8 shows the highest activity of the three −1 boxes for the TALEs with 40- and 42-amino-acid aberrant repeats ( Fig. 4b ). The TALE with a 30-amino-acid aberrant repeat has a similarly high activity with the −1 boxes deleted at position 8 and 9, respectively ( Fig. 4b ). This suggests that it is the aberrant repeat itself that is excluded in frameshift binding. 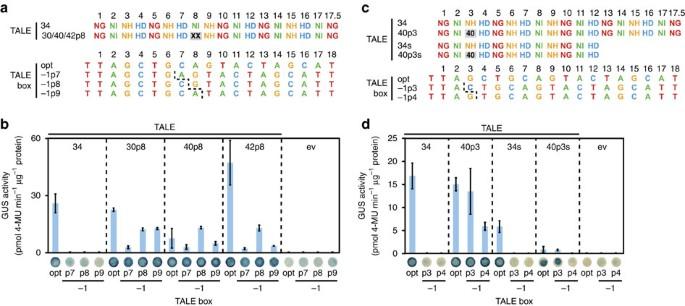Figure 4: Aberrant repeats allow recognition of target box frameshift close to their position. (a) RVDs of artificial TALEs and target boxes. A TALE with all 34-aa repeats or TALEs with an aberrant 30-aa NI-repeat, 40-aa NN-repeat and 42-aa NI-repeat, respectively, at position 8 are constructed. TALE boxes are either perfectly matching the specificity of normal repeats (opt) or have one base pair deleted to the right of the dashed line at position 7 (−1p7), position 8 (−1p8) or position 9 (−1p9). (b) GUS assays (n=3) of TALEs and reporter constructs described in (a). (b,d) 35S-driven GFP expression serves as empty vector (ev) control in quantitative and qualitative assays. Error bars indicate the s.d. in the quantitative assay. One representative leaf disk of the qualitative assay is shown. (c) TALE RVDs and target boxes. Artificial TALEs with either 17.5 or 11.5 repeats are constructed with a normal 34-aa NH-repeat or an aberrant 40-aa NN-repeat (grey box) inserted at position 3. The target boxes are either perfectly matching the specificity of normal repeats (opt) or have one base pair deleted to the right of the dashed line at position 3 (−1p3) or position 4 (−1p4). (d) GUS assays (n=3) of TALEs and reporter constructs described in (c). Figure 4: Aberrant repeats allow recognition of target box frameshift close to their position. ( a ) RVDs of artificial TALEs and target boxes. A TALE with all 34-aa repeats or TALEs with an aberrant 30-aa NI-repeat, 40-aa NN-repeat and 42-aa NI-repeat, respectively, at position 8 are constructed. TALE boxes are either perfectly matching the specificity of normal repeats (opt) or have one base pair deleted to the right of the dashed line at position 7 (−1p7), position 8 (−1p8) or position 9 (−1p9). ( b ) GUS assays ( n =3) of TALEs and reporter constructs described in ( a ). ( b , d ) 35S-driven GFP expression serves as empty vector (ev) control in quantitative and qualitative assays. Error bars indicate the s.d. in the quantitative assay. One representative leaf disk of the qualitative assay is shown. ( c ) TALE RVDs and target boxes. Artificial TALEs with either 17.5 or 11.5 repeats are constructed with a normal 34-aa NH-repeat or an aberrant 40-aa NN-repeat (grey box) inserted at position 3. The target boxes are either perfectly matching the specificity of normal repeats (opt) or have one base pair deleted to the right of the dashed line at position 3 (−1p3) or position 4 (−1p4). ( d ) GUS assays ( n =3) of TALEs and reporter constructs described in ( c ). Full size image To corroborate this finding, we use a TALE with a 40-amino-acid aberrant repeat placed at position 3 in either a 17.5 repeat or an 11.5 repeat array ( Fig. 4c ). It has been described that the initial repeats have a stronger impact on the overall TALE binding than later repeats [37] , [47] . Therefore, we reason that these TALEs will have a clear preference for the −1 box in which the nucleotide is missing that corresponds to the repeat that is excluded. The TALEs were combined with an optimal target box or boxes deleted in the nucleotide at position 3 or 4 ( Fig. 4c ). Indeed, the TALEs induce a higher reporter activity with the box carrying a −1 deletion at position 3 that corresponds to the position of the aberrant repeat than with the box with the deletion at position 4 ( Fig. 4d ). The shorter TALEs have a significantly weaker activity suggesting that the overall DNA recognition was partly compromised ( Fig. 4d ). In summary, we postulate that the aberrant repeat itself loops out of the repeat array when the TALE is bound to a target sequence with a single nucleotide deletion, but is inserted into the array when bound to an optimal box ( Fig. 7 ). Figure 7: Cartoons of repeat arrays in the normal and the looped-out conformation. Model of TALE repeats consisting of standard 34-aa repeats and repeat arrays containing one repeat of aberrant length, respectively, aligned to an optimal box or a −1 frameshift box. 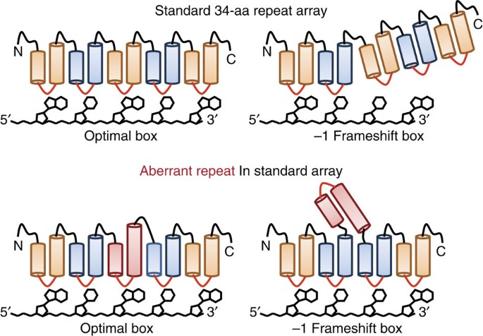Figure 7: Cartoons of repeat arrays in the normal and the looped-out conformation. Model of TALE repeats consisting of standard 34-aa repeats and repeat arrays containing one repeat of aberrant length, respectively, aligned to an optimal box or a −1 frameshift box. The aberrant repeat is shown in dark red. The aberrant repeat is shown in dark red. Full size image Tandem aberrant repeats are not flexible We analyse whether tandem aberrant repeats are accepted in a TALE repeat array. For this, we generate a TALE with aberrant 40-amino-acid repeats at position 8 and 9 in the frameshift-sensitive 17.5 repeat array used before ( Fig. 5a ). The TALE with the two aberrant repeats recognizes exclusively the box with a −1 frameshift at position 9 and neither the optimal one nor a −2 or +1 frameshift box ( Fig. 5b ). Apparently, the tandem aberrant repeats can only be compensated by one repeat being excluded from the interaction. This suggests that two neighbouring 40-amino-acid repeats can neither loop out simultaneously nor be arranged in the consecutive array of normal repeats. It cannot be excluded that aberrant repeats destabilize the TALE protein structure in certain repeat arrangements although we do not detect strong differences in protein amounts of the artificial TALEs used here and in the previous experiments with or without aberrant repeats, respectively ( Supplementary Fig. 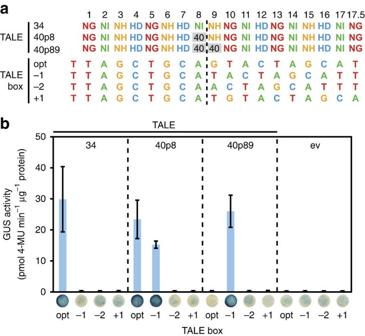6 ). Figure 5: Two aberrant repeats can be combined in tandem. (a) RVDs of artificial TALEs and target boxes. A TALE with all 34-aa repeats or TALEs with one or two 40-aa NN-repeats at position 8 (40p8) or 8 and 9 (40p89) are constructed. An optimal target box (opt) and derivatives with deletions of one or two nucleotides (−1 or −2) or an insertion of one nucleotide (+1) after position 8 (dashed line) are fused to a minimal promoter and a promoter-less GUS reporter gene. (b) GUS assays of TALEs and reporter constructs (n=3). 35S-driven GFP expression serves as empty vector (ev) control in quantitative and qualitative assays. Error bars indicate the s.d. in the quantitative assay. One representative leaf disk of the qualitative assay is shown. Figure 5: Two aberrant repeats can be combined in tandem. ( a ) RVDs of artificial TALEs and target boxes. A TALE with all 34-aa repeats or TALEs with one or two 40-aa NN-repeats at position 8 (40p8) or 8 and 9 (40p89) are constructed. An optimal target box (opt) and derivatives with deletions of one or two nucleotides (−1 or −2) or an insertion of one nucleotide (+1) after position 8 (dashed line) are fused to a minimal promoter and a promoter-less GUS reporter gene. ( b ) GUS assays of TALEs and reporter constructs ( n =3). 35S-driven GFP expression serves as empty vector (ev) control in quantitative and qualitative assays. Error bars indicate the s.d. in the quantitative assay. One representative leaf disk of the qualitative assay is shown. Full size image Aberrant repeats can participate in TALE–DNA recognition We want to clarify whether the RVD of the aberrant repeat participates in DNA base recognition when the TALE binds in the regular fashion to an optimal box. For this, we compare how TALEs with 34-amino-acid repeats and TALEs with an aberrant repeat deal with non-matching bases around the position of the aberrant repeat. We expect that a TALE with an aberrant repeat will display a reduced activity at the mismatch boxes if the RVD of the aberrant repeat participates in base recognition. TALEs with only 34-amino-acid repeats or an aberrant repeat of 30-, 40- or 42-amino-acid length, respectively, at position 8 are used. The aberrant repeat RVDs are NI or NN, which are compatible with the base adenine, but not thymine. We combine the TALEs with target boxes that contain 1–3 non-matching bases starting at position 8 or 9 ( Fig. 6a ). The TALE with normal 34-amino-acid repeats trigger significantly decreasing reporter activity with increasing number of mismatches ( Fig. 6b ). The TALEs with aberrant repeats show a very similar pattern. In particular, at the box with one mismatch at the position of the aberrant repeat (box 8.1; Fig. 6b ) reporter activity is significantly less than at the optimal one. This indicates that all tested aberrant repeats contribute to DNA–base recognition when the TALE binds an optimal box ( Fig. 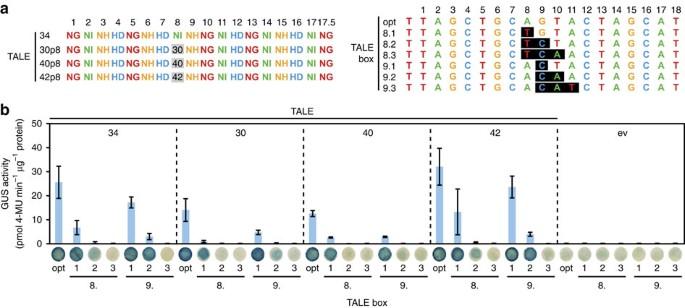7 ). Figure 6: Aberrant repeats participate in TALE–DNA base pair recognition. (a) TALE RVDs and target boxes. Artificial TALEs are constructed with all 34-aa repeats or aberrant repeats. An aberrant 30-aa NI-repeat, 40-aa NN-repeat and 42-aa NI-repeat is inserted at position 8, respectively. Target DNA boxes are either perfectly matching the specificity of normal repeats (opt) or have one to three non-matching bases (transversions) between position 8 and 11 (black boxes). (b) GUS assays of TALEs and reporter constructs (n=3). 35S-driven GFP expression serves as empty vector (ev) control in quantitative and qualitative assays. Error bars indicate the s.d. in the quantitative assay. One representative leaf disk of the qualitative assay is shown. Figure 6: Aberrant repeats participate in TALE–DNA base pair recognition. ( a ) TALE RVDs and target boxes. Artificial TALEs are constructed with all 34-aa repeats or aberrant repeats. An aberrant 30-aa NI-repeat, 40-aa NN-repeat and 42-aa NI-repeat is inserted at position 8, respectively. Target DNA boxes are either perfectly matching the specificity of normal repeats (opt) or have one to three non-matching bases (transversions) between position 8 and 11 (black boxes). ( b ) GUS assays of TALEs and reporter constructs ( n =3). 35S-driven GFP expression serves as empty vector (ev) control in quantitative and qualitative assays. Error bars indicate the s.d. in the quantitative assay. One representative leaf disk of the qualitative assay is shown. Full size image Aberrant repeats influence AvrXa7 and PthXo3 target range The natural aberrant repeats provide an extended flexibility to the repeat array that is not present in TALEs with standard repeats, and it is tempting to speculate that this has evolved to benefit Xanthomonas virulence. One possibility is that aberrant repeats enable Xanthomonas to recognize promoter variants in different plant cultivars or species. We investigate whether there are natural insertion/deletion (indel) mutations in the OsSWEET14 promoter region targeted by PthXo3. We compare this region in full genomic alignments of Oryza sativa japonica cv. Nipponbare, O. sativa indica , O. brachyantha and O. glaberrima . While we do not observe a difference between O. sativa japonica and O. sativa indica , we indeed find a single base-pair insertion at position 18/19 of the PthXo3 box in O. brachyantha , which may be compensated by the aberrant repeat of PthXo3 ( Supplementary Fig. 7 ). Interestingly, while binding of PthXo3 to its target box in O. sativa is preferred in the looped-out conformation (6 instead of 10 mismatches), binding in the normal conformation should be preferred in O. brachyantha (4 instead of 9 mismatches; Supplementary Fig. 7 ). To study the contribution of the aberrant repeat in the natural TALE AvrXa7 on target recognition, we assemble an artificial TALE with the same RVD composition as AvrXa7 (termed ArtXa70) and a derivative (ArtXa71) with a normal 34-amino-acid repeat instead of the aberrant 39-amino-acid-repeat at position 13 ( Supplementary Fig. 8a,b ). Both artificial TALEs recognize the optimal box in GUS assays similarly well as AvrXa7, but the TALE without the aberrant repeat (ArtXa71) is significantly compromised on the −1 target box ( Supplementary Fig. 8c ). This indicates that the aberrant repeat also contributes to the flexible target box recognition of the natural TALE AvrXa7 ( Supplementary Fig. 1 ). TALEs with aberrant repeats can break plant resistance To test whether TALEs with aberrant repeats contribute to bacterial virulence, we design TALEs based on a naturally occurring promoter allele that confers plant resistance. Rice Xa25 ( Os-SWEET13 ) encodes a SWEET protein that supports Xanthomonas virulence probably facilitated by the TALE PthXo2 (refs 16 , 19 ). A natural single base-pair insertion mutation in the recessive xa25 allele results in plants resistant to Xoo likely by prohibiting binding of PthXo2, which does not contain any aberrant repeats [17] ( Supplementary Fig. 9a ). To test whether TALEs with aberrant repeats can overcome this resistance, we construct TALEs targeting the PthXo2-binding site in the recessive xa25 allele either with 17.5 exclusively regular 34-amino-acid repeats (ArtXa251, Fig. 8 and Supplementary Fig. 9b ) or one aberrant repeat at position 4 (ArtXa252, Fig. 8 and Supplementary Fig. 9c ). The xa25 and Xa25 promoter regions are cloned from O. sativa cv. Nipponbare and O. sativa cv. Zhenshan 97, respectively [17] . Agrobacterium-mediated production of ArtXa251 triggers reporter gene activation of the xa25 (Nipponbare; that is, optimal box), but not the Xa25 (Zhenshan 97; that is, −1 frame-shift box) promoter ( Supplementary Fig. 9d ), supporting that normal TALEs are highly compromised by indel mutations. In contrast, the TALE with an aberrant repeat, ArtXa252, induces expression of both reporter constructs ( Supplementary Fig. 9d ). 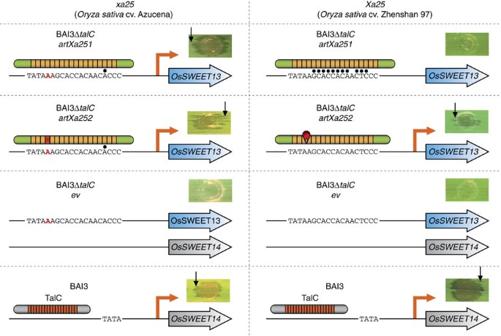Figure 8: TALEs with aberrant repeat can overcome plant resistance. Disease phenotypes ofXanthomonas oryzaepv.oryzae(Xoo) strains onOryza sativaleaves. Leaves of 3–4 week-old Azucena or Zhenshan 97 plants are inoculated with strain BAI3 or BAI3ΔtalCcarrying empty vector (ev) or TALEartXa251orartXa252. Pictures are taken 4 days post inoculation. Azucena and Zhenshan 97 contain alleles ofOsSWEET13, termedxa25andXa25, respectively, which differ in their promoter sequences by an additional nucleotide (red). The strain harbouring ArtXa252 with a 40-aa repeat (red) causes water soaking disease symptoms (black arrows) on both alleles. Black dots indicate RVD–base -mismatches. The experiments are performed twice with similar results. Figure 8: TALEs with aberrant repeat can overcome plant resistance. Disease phenotypes of Xanthomonas oryzae pv. oryzae ( Xoo ) strains on Oryza sativa leaves. Leaves of 3–4 week-old Azucena or Zhenshan 97 plants are inoculated with strain BAI3 or BAI3Δ talC carrying empty vector ( ev ) or TALE artXa251 or artXa252 . Pictures are taken 4 days post inoculation. Azucena and Zhenshan 97 contain alleles of OsSWEET13 , termed xa25 and Xa25 , respectively, which differ in their promoter sequences by an additional nucleotide (red). The strain harbouring ArtXa252 with a 40-aa repeat (red) causes water soaking disease symptoms (black arrows) on both alleles. Black dots indicate RVD–base -mismatches. The experiments are performed twice with similar results. Full size image We further analyse the contribution of TALEs with aberrant repeats to Xanthomonas spp. infections. The Xoo strain BAI3 causes disease on rice cultivars Azucena and Zhenshan 97 in part because it contains the TALE TalC that directs expression of the gene encoding the sugar exporter OsSWEET14 (ref. 21 ) ( Fig. 8 ). Deletion of talC renders the bacteria unable to cause disease [21] ( Fig. 8 ), but this can be compensated by artificial TALEs that trigger expression of OsSWEET13 (ref. 19 ). We introduce ArtXa251 and ArtXa252 into Xoo BAI3Δ talC and infect rice cultivars Azucena ( xa25 ) and Zhenshan 97 ( Xa25 ), which differ in their OsSWEET13 promoter region by the 1-bp indel mutation ( Fig. 8 ). The Xoo strain containing ArtXa251 with exclusively normal repeats causes disease symptoms on O. sativa cv. Azucena, but not O. sativa cv. Zhenshan 97 ( Fig. 8 ), because of the indel mutation in the target box. In contrast, Xoo containing ArtXa252 with the aberrant repeat causes disease symptoms on both rice cultivars ( Fig. 8 ). This demonstrates that aberrant repeats can enable Xanthomonas to compensate for indels in target promoters and break natural plant resistances. Apparently, aberrant repeats are an evolutionary solution for Xanthomonas spp. to overcome small indel mutations that otherwise efficiently block TALE binding. We have described an exceptional and surprising recognition pattern of TALEs that has implications for the general concept of TALE–DNA interaction as well as the evolutionary adaptation of these important virulence factors. The near-identical amino-acid sequence of Xanthomonas TALE repeats implies that this regularity is required for binding to the highly symmetric structure of the DNA double helix [9] , [10] , [14] . Nevertheless, in nature the glycine and the leucine at positions 14 and 29, respectively, are the only amino acids conserved in all TALE repeat sequences [5] . Even more striking are natural repeat variants that deviate from the typical 34- or 35-amino-acid length of TALE repeats, because they are expected to impose a structural problem to the overall repeat array. Here, we show that either shorter (30 amino acids) or longer repeat variants (39, 40 or 42 amino acids) change the DNA-binding behaviour of TALEs. They can either insert into the repeat array like normal repeats or be excluded from the interaction to facilitate a shift of the following repeats forward by one position depending on the best fit of all RVDs to a given target sequence ( Figs 2 and 7 ). This behaviour is not possible for TALEs with normal 34-amino-acid repeats. In the absence of structural data, we favour a model that the aberrant repeat loops out of the repeat array, because this seems to be sterically the easiest solution; alternative scenarios are possible though. Surprisingly, all aberrant repeats tested functioned in a comparable way although we have not compared them in all assays in our study. In part this might be explained by the fact that the aberrant repeat sequences are all related to a normal 34-amino-acid TALE repeat. They contain either a short deletion in the second α-helix (30-amino-acid repeat) or a duplicated first (42-amino-acid repeat) or second α-helix (39/40-amino-acid repeats) flanking the RVD ( Fig. 1 ). Possibly, these duplications of structural elements still allow the hydrophobic repeat-to-repeat interactions that stabilize the normal repeat array [9] , [10] . At the same time, the aberrant repeats probably do not fit perfectly into the array, thereby weakening inter-repeat interactions and causing a local flexibility and structural tension that allows the aberrant repeat to loop out. In general, TALEs exhibit a highly flexible structure. Molecular dynamics simulations show that the TALE repeat region has a high conformational plasticity [48] . In addition, structural data and computational simulations indicated that the TALE repeat superstructure condenses upon interaction with cognate DNA resulting in more densely packed repeats than in the DNA-free form [9] , [41] , [48] . Likely, the flexible nature of the repeat region allows the unique binding mode conferred by aberrant repeats. How does an aberrant repeat influence the dynamics of TALE protein–DNA interaction? Insertion of aberrant repeats in the rear part of the repeat array compromised TALE-mediated gene induction in our experiments ( Fig. 3 ). We postulate that the aberrant repeat weakens the protein–DNA interaction and that a minimum number of repeats following the aberrant one is required to allow subsequent condensation of the rear repeats onto the DNA double helix. The N-terminal domain of TALEs mediates unspecific interaction to DNA as well as recognition of the initial thymine [7] , [8] , [10] . In addition, the initial repeats after the N-terminal domain are more important for binding than downstream repeats [37] , [47] . Together, these observations support a model where the N-terminal TALE region scans the DNA and the repeats subsequently condense at target sequences onto the DNA in a consecutive fashion starting from the N-terminal region. Possibly, an aberrant repeat that is excluded from binding in a frameshift scenario only allows condensation of further repeats, if their number is sufficiently high to condense onto the DNA in a separate event. Accordingly, the aberrant repeat might separate the repeat domain into two binding domains. In general, the tolerance of aberrant repeats in a repeat array likely depends on the overall binding energies of preceding and following repeats. Surprisingly, two tandem aberrant repeats only recognize a −1 frameshift box and not a normal one nor a −2 frameshift box ( Fig. 5 ). This implies that the loop out conformation has specific requirements and does not allow looping out of more than one repeat. Furthermore, the additional structural perturbation of two near aberrant repeats does not allow a normal repeat arrangement. It is presently difficult to estimate how many aberrant repeats may be accepted in a TALE repeat domain. The novel binding mode comprises interesting potential for biotechnology applications that are otherwise difficult to achieve. TALEs and TALENs with aberrant repeats can be used to simultaneously recognize allelic variants that differ by single nucleotide frameshifts. For synthetic TALE biology [49] , master regulators with aberrant repeats might be used to control two subsets of target sequences that differ by indel mutations. This is difficult to achieve with CRISPR/Cas9 recognition of DNA sequences, because its RNA-guided recognition mechanism cannot compensate for indel mutations [50] . In addition, it is tempting to speculate that the aberrant repeats can function as an insertion point for more complex peptide tags or proteins within the TALE repeat domain to generate unique fusion proteins. A significant aspect of our study is that these aberrant repeats are naturally evolved variants. Their presence in important virulence factors implies that they confer a selective advantage. The battle between pathogen and host is characterized by a constant struggle for innovation and counteracting activities to prevent losing the evolutionary race. Inherently, TALEs are especially sensitive to frameshift mutations in their target sequence and this has been exploited by natural plant resistances [16] , [20] , [25] . An aberrant repeat contributes a new degree of flexibility to the DNA-binding activity of a TALE without strong penalty on overall activity. We showed that TALEs with aberrant repeats can enable Xoo to overcome a natural resistance that is caused by a 1-bp deletion. As another example, the aberrant repeat in PthXo3 and AvrXa7 might have evolved to recognize unknown target box variants in response to a specific mutation that occurred in the OsSWEET14 promoter in some rice cultivars. Alternatively, our computational search of available OsSWEET14 promoter sequences raises the possibility that this potent virulence factor might favour colonization of Xoo on the different rice species O. sativa and O. brachyantha . So far, the possibility that TALEs of one bacterial strain support virulence in different host species has not been explored, but it is typical for type III effectors that they function in different plants and even non-plants [51] , [52] . Further analysis of natural TALEs with aberrant repeats and their target promoters will clarify the role of these unique virulence factors for the pathogen. Our data reveal that designer resistances based on mutations in TALE target boxes [16] have to be considered carefully to be effective. Bacterial strains and growth conditions Xanthomonas oryzae pv. oryzae ( Xoo ) BAI3 and BAI3Δ talC are used in this study [21] , [53] . Plasmids are introduced into Xoo by conjugation using pRK2013 as a helper plasmid in triparental matings [54] . Rifampicin (100 μg ml −1 ) and gentamicin (20 μg ml −1 )-resistant clones are selected upon plating on PSA medium and one isolate is chosen for further experiments. Escherichia coli is cultivated at 37 °C in lysogeny broth and Agrobacterium tumefaciens GV3101 at 30 °C in yeast extract broth supplemented with appropriate antibiotics. Plant growth and inoculations Nicotiana benthamiana plants are cultivated in the greenhouse with 16 h light, 40–60% humidity and day/night temperatures of 23 °C/19 °C. Plants inoculated with Agrobacterium strains are transferred to a Percival growth chamber (Percival Scientific) with 22 °C/18 °C day/night temperatures and 16 h light. Rice experiments are performed under greenhouse conditions with cycles of 12 h of light at 26 °C, 70% relative humidity and 12 h of dark at 25 °C, 70% relative humidity. Oryza sativa subsp. japonica cv. Azucena and O. sativa subsp. indica cv. Zhenshan 97 are used for virulence assays. Leaves of 3–4-week-old plants are infiltrated with a bacterial suspension at an optical density of 0.5 at 600 nm (OD 600 ) using a needle-less syringe [55] . Pictures from disease symptoms (water-soaked lesions) are taken 4 days post inoculation. Construction of repeat modules with aberrant repeats Primer pairs encoding natural repeats of aberrant length are designed such that forward and reverse primer overlap in their 3′ part ( Supplementary Tables 1 and 3 ). Phusion polymerase is used to extend the primers and the resulting DNA fragments are subcloned into pUC57 via SmaI cut-ligation. The resulting plasmids are used as template to amplify the aberrant repeats with primers that add BpiI restriction sites matching the existing Golden TAL Technology kit to insert the aberrant repeats at position 2 or 3 into a hexa-repeat array [46] . Construction of artificial TALEs TALEs are constructed using the Golden TAL Technology [46] . Up to six individual repeats with selected RVDs are subcloned in an assembly vector. To construct AvrXa7-derivatives with 25.5 repeats, we extend the original Golden TAL kit [46] with two novel assembly vectors ( Supplementary Note 1 ). The repeat backbone apart from the RVDs is identical ( Supplementary Table 4 ). The repeats are pre-assembled in 2–5 assembly vectors and inserted together with the Hax3 N- and C-terminal regions [56] . For expression in planta , N-terminal GFP–TALE fusion are assembled in a Golden Gate-compatible binary vector allowing expression of the constructs under control of the constitutive 35S promoter. For examples of DNA and amino-acid sequences see Supplementary Note 1 . For expression in Xanthomonas spp., TALE–FLAG fusions are assembled in a Golden Gate-compatible broad host range vector [19] . GUS reporter constructs and reporter assay OsSWEET13 ( Xa25 / xa25 , Os12N3 and Os12g29220 ) 1 kb promoter fragments ( Supplementary Note 1 ), an OsSWEET14 ( Os11N3 and Os11g31190 ) 341-bp promoter fragment, and artificial and natural TALE boxes ( Supplementary Table 3 ) together with the minimal Bs4 promoter, respectively, are inserted into pENTR/D-TOPO (Invitrogen). The promoter derivatives are recombined into pGWB3 (ref. 57 ) via LR recombination. Transient GUS reporter assays are performed [7] . Briefly, Agrobacterium strains delivering TALE constructs and GUS reporter constructs are mixed 1:1 and inoculated into leaves of 5–7-week-old N. benthamiana plants with a total OD 600 of 0.8. The T-DNAs integrate into the plant chromosomes. Leaf disks (0.9 cm diameter) are sampled 2 days later and GUS activity is determined. For qualitative GUS assays, leaf disks are stained in X-Gluc (5-bromo-4-chloro-3-indolyl-β- D -glucuronide) solution, destained in ethanol and dried between acetate foil. For quantitative GUS assays two leaf disks are pooled, the plant tissue homogenized, diluted and incubated with 4-methyl-umbelliferyl-β- D -glucuronide (MUG). Proteins are quantified using Bradford assay (Roth). Values from three plants are combined into one data point. All experiments are done at least twice with similar results. Construction of TALENs TALENs are constructed from modules matching the Golden TAL Technology [46] . The repeats are assembled in hexa-repeat modules and inserted together with modified short N- and C-terminal modules into a compatible ENTRY vector (pEGG). The N-terminal TALEN module contains amino acids 153–288 of Hax3, a SV40 nuclear localization sequence, and a tag (c-myc-tag for forward TALEN and FLAG-tag for reverse TALEN) sequence (see Supplementary Note 1 ). The C-terminal TALEN module contains amino acids 1–63 of the C-terminal region of Hax3 and a heterodimeric (DS for forward TALEN and RR for reverse TALEN) ‘sharkey’ Fok I endonuclease domain [58] . The TALEN are transferred via GATEWAY (Invitrogen) LR recombination into pDEST17 under control of a T7 promoter. TALEN in vitro cleavage assay TALENs are expressed using the TnT T7 Quick Coupled Transcription/Translation System (Promega) following the manufacturer’s instructions. Five hundred nanograms of DNA from each TALEN construct are used. The target DNA fragment is generated by linearization of pENTR containing the respective target box upstream of the minimal Bs4 promoter using the restriction enzyme Alw 44I (Thermo Scientific) following the manufacturer’s instructions and subsequent purification with the GeneJET PCR Purification Kit (Thermo Scientific). For the in vitro cleavage assay 4 μl of TnT reaction containing the TALEN pair proteins is mixed with 200 ng of target DNA in 1 × NEBuffer 3 (New England Biolabs) supplied with 2.5 μg μl −1 BSA to a total volume of 20 μl. After incubation for 60 min at 37 °C the reaction is inactivated at 65 °C for 20 min and centrifuged at 16,000 g for 3 min. The supernatant (16 μl) is analysed on a 1% agarose gel. All experiments are at least done twice with similar results. Immunoblotting For plant immunoblotting TALEs are transiently expressed in N. benthamiana for 2 days. Agrobacterium strains are inoculated with an OD 600 of 0.4. Two leaf disks are pooled, the plant tissue homogenized, resuspended in 90 μl Lämmli buffer and incubated at 95 °C for 10 min. Debris are pelleted and SDS-PAGE is performed with 15 μl of each sample. The proteins are transferred to a PROTRAN nitrocellulose membrane (Whatman). To detect GFP-tagged proteins membranes are incubated with anti-GFP rabbit serum (Life Technologies; dilution 1:2,000). For detection by enhanced chemiluminescence (ECL) ECL anti-rabbit IgG (GE Healthcare; dilution 1:10,000) is used. How to cite this article: Richter, A. et al. A TAL effector repeat architecture for frameshift binding. Nat. Commun. 5:3447 doi: 10.1038/ncomms4447 (2014).